Evolution of a tissue-specific silencer underlies divergence in the expression ofpax2andpax8paralogues Recent studies underscore a role for the differential degeneration of enhancers in the evolutionary diversification of paralogue expression. However, no one has reported evidence for the involvement of innovative cis -regulatory changes. Here we show that silencer innovation diversified expression of the vertebrate paralogues, pax2 and pax8 . pax2 shows multi-tissue expression, as does the ancestral amphioxus orthologue, pax2/5/8 , whereas pax8 expression localizes to a subset of pax2 -expressing tissues. We reveal that both pax2 and pax8 retain ancestral enhancers capable of directing pax2 -like, multi-tissue expression. However, a silencer within the pax8 proximal promoter suppresses pleiotropic enhancer activity outside the pax8 -expressing tissues. In contrast, the combination of the pax2 proximal promoter with either the pax8 or pax2 enhancer recapitulates pax2 -like expression, as in the amphioxus pax2/5/8 promoter. We propose that silencer innovation, rather than enhancer degeneration, was crucial for the divergent expression of paralogues with pleiotropic enhancers inherited from their common progenitor. During chordate evolution, two rounds of whole-genome duplication (WGD1 and WGD2) occurred in the vertebrate ancestor, to be followed later by a third round (WGD3) in the teleost lineage [1] , [2] . These WGDs generated a number of duplicated gene pairs (known as paralogues) from the ancestral gene set, with members of sibling paralogues often showing overlapping, yet distinct, expression patterns in modern vertebrates. The evolutionary mechanisms underlying this divergence of expression can be explained by the duplication–degeneration–complementation model [3] . This model is based on the regulatory complexity of developmental genes that generally have an array of multiple enhancers for discrete expression domains. It assumes that degenerative mutations occur much more frequently than do innovative ones. The model predicts that, after the WGD(s), parts of duplicated enhancers were lost reciprocally from sibling paralogues because of degenerative mutations, but at least one enhancer copy will remain in either of the paralogues so that their resulting complementary expressions cover the original full expression of the progenitor gene, a process known as subfunctionalization. This model is supported by discoveries of complementary enhancer degeneration in teleost paralogues generated by WGD3 [4] , [5] . For example, the mammalian Pax6 gene has multiple cis -regulatory elements, including enhancers for the pancreas, telencephalon and diencephalon [6] . These enhancers are conserved in tetrapods, but were lost reciprocally from the duplicated zebrafish pax6 genes because of degenerative mutations: one lost the pancreas enhancer and the other lost the telencephalon and diencephalon enhancers. However, although the WGDs are expected to have stimulated not only such degenerative cis -regulatory changes but also innovative changes, involvement of the latter phenomena—such as enhancer and/or silencer acquisition—remains unknown. In addition, it is unclear to what extent such degenerative cis -regulatory changes can account for the divergence in the expression of paralogues generated by the earlier WGDs (WGD1 and WGD2), whose cis -regulatory changes are generally thought to have been more significant than those in the teleost-specific paralogues. The paired-domain transcription factor genes, pax8 and pax2 , are essential for the development of multiple organs, including the kidney [7] , [8] . These two genes and another related gene, pax5 , arose from a single progenitor following WGD1 and WGD2 [9] , [10] , [11] . Pax8 is mainly expressed in the kidney, ear and thyroid gland during development [12] , [13] , while pax2 shows expression not only in the pax8 -expression domains but also in other tissues such as the eye, pharyngeal arches, midbrain–hindbrain boundary (MHB), hindbrain and spinal cord [14] , [15] . The cephalochordate amphioxus, which diverged from the vertebrate lineage before the WGDs occurred and likely retains ancestral modes of gene regulation, possesses the single orthologue, pax2/5/8 [9] . This gene shows pleiotropic expression in most of the tissues that are homologous to the vertebrate pax2 -expressing tissues, implying that pax2 retains most of the ancestral regulatory mechanisms. In this study, we chose pax8 , pax2 and pax2/5/8 as models for investigating regulatory diversification after WGD1 and WGD2. We found that both pax8 and pax2 have inherited ancestral enhancers from their common progenitor and that silencer innovation within the pax8 proximal promoter, rather than enhancer degeneration, accounts for the divergent expression of this paralogue pair. This is the first evidence for the involvement of an innovative cis -regulatory change in the evolutionary diversification of paralogue expression. Conserved non-coding sequences in pax8 and pax2 loci To explore the cis -regulatory evolution of pax8 and pax2 , we initially compared the genomic sequence of a 160-kb segment encompassing the human PAX8 gene with the orthologous interval in mouse, frog ( Xenopus tropicalis ) and pufferfish ( Takifugu rubripes ) genomes using the MultiPipMaker alignment tool [16] . This analysis identified five conserved non-coding sequences (CNSs), CNS1–CNS5, as candidates for pax8 enhancers ( Fig. 1a ; Supplementary Fig. S1 ). CNS1 and CNS2 are conserved from the human to pufferfish, whereas CNS3–CNS5 are found only in tetrapods. We also compared the pax8 genomic sequences with the genomic sequences from the human, mouse, frog and pufferfish pax2 loci, and found the conservation of a recognizable paralogous sequence of pax8 CNS1 ( pax8 -CNS1) in the 5′-flanking region of pax2 ( Fig. 1a ; Supplementary Fig. S1 ). Local alignment of such duplicated sequences, pax8 -CNS1 and pax2 -CNS1, revealed the conservation of a cluster of putative transcription factor-binding motifs ( Fig. 1b ). This finding implies partial conservation of ancestral regulatory mechanisms between pax8 and pax2 , which might account for their overlapping expression in the pronephros and otic vesicle during embryonic development ( Fig. 1c,d ). 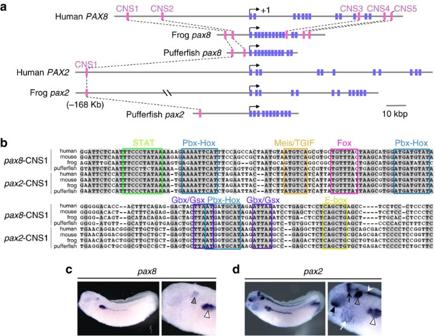Figure 1: The CNSs and embryonic expression ofpax8andpax2. (a) Diagram of vertebratepax8andpax2loci showing the position of CNSs. Magenta and purple boxes indicate CNSs and exons, respectively. Forpax2, onlypax2-CNS1—paralogous topax8-CNS1—is shown. Broken lines indicate orthologous and paralogous relationships between CNSs. CNS lengths range from 123 to 407 bp in the frog genome. (b) Alignment ofpax8-CNS1 andpax2-CNS1 sequences from the human, mouse, frog and pufferfish. Only their conserved core regions are shown. Nucleotides identical in more than six sequences are shaded in grey. Conserved transcription factor-binding motifs are boxed, although their functional significance was not examined in this study. (c,d)In situhybridization analysis showing expression ofpax8(c) andpax2(d) inX. tropicalistailbud embryos (stage 30). White, grey and black triangles indicate expression in the pronephros, otic vesicle and eye, respectively. White and black arrows indicate expression in the pharyngeal arches and MHB, respectively. A white arrowhead indicates expression in the hindbrain. Note that the thyroid gland expression ofpax2occurs later, from stage 3413. Figure 1: The CNSs and embryonic expression of pax8 and pax2 . ( a ) Diagram of vertebrate pax8 and pax2 loci showing the position of CNSs. Magenta and purple boxes indicate CNSs and exons, respectively. For pax2 , only pax2 -CNS1—paralogous to pax8 -CNS1—is shown. Broken lines indicate orthologous and paralogous relationships between CNSs. CNS lengths range from 123 to 407 bp in the frog genome. ( b ) Alignment of pax8 -CNS1 and pax2 -CNS1 sequences from the human, mouse, frog and pufferfish. Only their conserved core regions are shown. Nucleotides identical in more than six sequences are shaded in grey. Conserved transcription factor-binding motifs are boxed, although their functional significance was not examined in this study. ( c , d ) In situ hybridization analysis showing expression of pax8 ( c ) and pax2 ( d ) in X. tropicalis tailbud embryos (stage 30). White, grey and black triangles indicate expression in the pronephros, otic vesicle and eye, respectively. White and black arrows indicate expression in the pharyngeal arches and MHB, respectively. A white arrowhead indicates expression in the hindbrain. Note that the thyroid gland expression of pax2 occurs later, from stage 34 [13] . Full size image pax8 enhancers direct pax2 -like pleiotropic expression In the functional analysis, we first focused on the cis -regulatory landscape of pax8 . The Xenopus laevis system was chosen to examine the potential enhancer activity of the CNSs, because an efficient transgenesis technique for a non-mosaic founder assay is readily available [17] . Each X. tropicalis pax8 -CNS was cloned into a green fluorescent protein (GFP) reporter plasmid carrying a β -actin basal promoter [18] . Each construct was then used to generate transgenic embryos, and their GFP expression was examined once the resulting embryos reached the tailbud stages (stages 30–32) [19] . The reporter constructs without a CNS showed no significant GFP expression ( Fig. 2a ). By contrast, the constructs carrying pax8 -CNS1, pax8 -CNS2, pax8 -CNS3 or pax8 -CNS4, but not that carrying pax8 -CNS5, drove reproducible expression not only in the pronephros that expresses endogenous pax8 but also in other tissues that do not express pax8 at the developmental stages examined ( Fig. 2b–f , compare with Fig. 1c ; group pictures of transgenic embryos, scoring results and expression patterns are summarized in Supplementary Fig. S2 , and Supplementary Tables S1 and S2 , respectively). These tissues include the eye, pharyngeal arches, MHB and hindbrain, which are the pax2 -expression domains ( Fig. 1d ). Moreover, when all the pax8 -CNSs were assembled in a single reporter construct, its expression mostly recapitulated that of pax2 ( Fig. 2g ). Similar pax2 -like, pleiotropic expression was observed when the β -actin promoter of this construct was replaced with a β -globin basal promoter [20] ( Fig. 2h,i ), which indicated that pax2 -like expression patterns depend absolutely on the enhancer activity of the pax8 -CNSs. 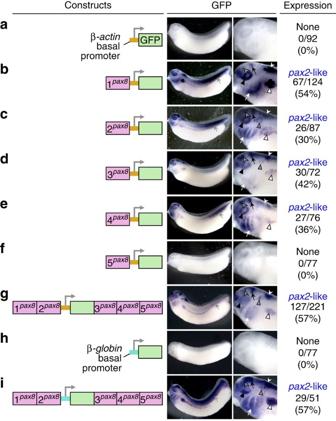Figure 2: GFP expression driven bypax8-CNSs recapitulates the pleiotropic expression ofpax2. TransgenicX. laevisembryos were generated with the following reporter constructs and their expression was analysed usingin situhybridization. (a) The β-actinbasal promoter alone was linked to GFP. (b–f) The β-actinpromoter-GFP cassette was flanked by eitherX. tropicalis pax8-CNS1 (b),pax8-CNS2 (c),pax8-CNS3 (d),pax8-CNS4 (e) orpax8-CNS5 (f). (g) The β-actinpromoter-GFP cassette was flanked by all thepax8-CNSs. (h) The β-globinbasal promoter alone was linked to GFP. (i) The β-globinpromoter-GFP cassette was flanked by all thepax8-CNSs. TheX. tropicalis pax8-CNS1 topax8-CNS5 are shown as 1pax8to 5pax8. Representative examples of GFP expression are shown together with the injected reporter constructs. The right-hand panels show high-magnification views of the embryonic head regions illustrated in the left-hand panels. GFP expression patterns are summarized on the extreme right with the scoring results. Numbers of embryos with the positive expression similar to the representative examples, and the total number of analysed embryos injected with each construct are indicated with percentages of the former cases. White, grey and black triangles indicate expression in the pronephros, otic vesicle and eye, respectively. White, grey and black arrows indicate expression in the pharyngeal arches, somites and MHB, respectively. White and grey arrowheads indicate expression in the hindbrain and anterior midbrain, respectively. Figure 2: GFP expression driven by pax8 -CNSs recapitulates the pleiotropic expression of pax2 . Transgenic X. laevis embryos were generated with the following reporter constructs and their expression was analysed using in situ hybridization. ( a ) The β -actin basal promoter alone was linked to GFP. ( b – f ) The β -actin promoter-GFP cassette was flanked by either X. tropicalis pax8 -CNS1 ( b ), pax8 -CNS2 ( c ), pax8 -CNS3 ( d ), pax8 -CNS4 ( e ) or pax8 -CNS5 ( f ). ( g ) The β -actin promoter-GFP cassette was flanked by all the pax8 -CNSs. ( h ) The β -globin basal promoter alone was linked to GFP. ( i ) The β -globin promoter-GFP cassette was flanked by all the pax8 -CNSs. The X. tropicalis pax8 -CNS1 to pax8 -CNS5 are shown as 1 pax8 to 5 pax8 . Representative examples of GFP expression are shown together with the injected reporter constructs. The right-hand panels show high-magnification views of the embryonic head regions illustrated in the left-hand panels. GFP expression patterns are summarized on the extreme right with the scoring results. Numbers of embryos with the positive expression similar to the representative examples, and the total number of analysed embryos injected with each construct are indicated with percentages of the former cases. White, grey and black triangles indicate expression in the pronephros, otic vesicle and eye, respectively. White, grey and black arrows indicate expression in the pharyngeal arches, somites and MHB, respectively. White and grey arrowheads indicate expression in the hindbrain and anterior midbrain, respectively. Full size image Tissue-specific silencing by the pax8 proximal promoter The discrepancy between the pleiotropic expression driven by the conserved pax8 enhancers and the more restricted expression of endogenous pax8 suggests the presence of a tissue-specific silencer(s) that limits enhancer function. As the tissue-specific expression pattern of pax8 is mostly conserved in vertebrates [11] , [13] , this silencer activity is also expected to be conserved evolutionarily. However, no conserved regions other than CNS1–CNS5 were found near the pax8 locus. Therefore, the proximal promoter region was examined for conserved regulatory function without apparent cross-species sequence conservation, as in the in vivo analysis of the PHOX2B gene combined with the in vitro data from the ENCODE project [21] . When the proximal promoter region of X. tropicalis pax8 (nucleotides −2038 to +130) alone was linked to GFP, no significant expression was observed ( Fig. 3a ). When this proximal promoter region was flanked by the Xenopus pax8 -CNS1 to pax8 -CNS5, GFP expression was observed only in the pronephros, hindbrain and a small anterior part of the midbrain, making a striking contrast to the pleiotropic expression driven by the β -actin and β -globin basal promoters flanked by the same set of pax8 -CNSs ( Fig. 3b , compare with Fig. 2g,i ). These results suggested that the pax8 promoter harboured tissue-specific silencer activity, which partly explains the restriction of the enhancer function to the correct expression domains of pax8 , such as the pronephros. Given that endogenous pax8 was not expressed in the hindbrain and midbrain but did show expression in the otic vesicle at the stages examined ( Fig. 1c ), pax8 may have another silencer and enhancer for these tissues. This possibility is also supported by a reporter assay using a fosmid construct that covers the −24 kb to +12 kb region of pax8 and faithfully recapitulates endogenous pax8 expression ( Supplementary Fig. S3 ). Deletion assays narrowed down the sequence responsible for the silencer activity to a 344-bp region (−214 to +130) in the proximal promoter ( Fig. 3c,d ). This 344-bp sequence suppressed the expression from heterologous promoters in an orientation- and distance-independent manner ( Supplementary Fig. S4 ), satisfying the criteria for a silencer [22] . 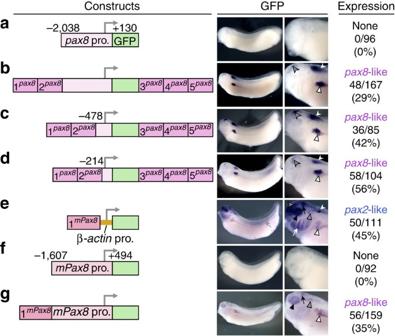Figure 3: Identification of tissue-specific silencer activity associated with thepax8proximal promoter. TransgenicX. laevisembryos were generated with the following GFP constructs. (a) The proximal promoter region ofX. tropicalis pax8(−2038 to +130) alone was linked to GFP. (b–d) A deletion series of theX. tropicalis pax8proximal promoter (b, −2038 to +130;c, −478 to +130; andd, −214 to +130) was flanked by theX. tropicalis pax8-CNS1 topax8-CNS5. (e) The mousePax8-CNS1 (shown as 1mPax8) was linked to the β-actinbasal promoter-GFP cassette. (f) The proximal promoter region of mousePax8(−1607 to +494) alone was linked to GFP. (g) The mousePax8proximal promoter was flanked by mousePax8-CNS1. White, grey and black triangles indicate expression in the pronephros, otic vesicle and eye, respectively. White, grey and black arrows indicate expression in the pharyngeal arches, somites and MHB, respectively. White and grey arrowheads indicate expression in the hindbrain and an anterior part of the midbrain, respectively. Figure 3: Identification of tissue-specific silencer activity associated with the pax8 proximal promoter. Transgenic X. laevis embryos were generated with the following GFP constructs. ( a ) The proximal promoter region of X. tropicalis pax8 (−2038 to +130) alone was linked to GFP. ( b – d ) A deletion series of the X. tropicalis pax8 proximal promoter ( b , −2038 to +130; c , −478 to +130; and d , −214 to +130) was flanked by the X. tropicalis pax8 -CNS1 to pax8 -CNS5. ( e ) The mouse Pax8 -CNS1 (shown as 1 mPax8 ) was linked to the β -actin basal promoter-GFP cassette. ( f ) The proximal promoter region of mouse Pax8 (−1607 to +494) alone was linked to GFP. ( g ) The mouse Pax8 proximal promoter was flanked by mouse Pax8 -CNS1. White, grey and black triangles indicate expression in the pronephros, otic vesicle and eye, respectively. White, grey and black arrows indicate expression in the pharyngeal arches, somites and MHB, respectively. White and grey arrowheads indicate expression in the hindbrain and an anterior part of the midbrain, respectively. Full size image The functional cross-species conservation of both the pleiotropic enhancer and the proximal promoter-associated silencer was examined using the sequences from the mouse Pax8 locus. As expected from sequence conservation, mouse Pax8 -CNS1 drove pax2 -like, multi-tissue expression from the β -actin promoter in Xenopus embryos as with the Xenopus pax8 -CNS1 ( Fig. 3e ). A proximal promoter region of mouse Pax8 (−1607 to +494) in itself drove no significant GFP expression, as with the Xenopus pax8 proximal promoter ( Fig. 3f ). When this mouse Pax8 promoter was flanked by the mouse Pax8 -CNS1, GFP expression was observed only in the pronephros, otic vesicle, MHB and eye ( Fig. 3g ), indicating tissue-specific suppression of enhancer activity by the promoter. Note that mouse Pax8 exhibits expression not only in the pronephros and otic vesicle but also in the MHB [8] , in contrast to Xenopus pax8 that does not exhibit expression in the MHB [13] ( Fig. 1c ). Thus, GFP expression driven by the mouse Pax8 -CNS1 from the mouse Pax8 proximal promoter mostly recapitulated the mouse Pax8 expression in Xenopus embryos, although the ectopic expression remaining in the eye suggests the presence of another silencer in mouse Pax8 . Enhancer conservation and silencer innovation The comparative genome sequence analysis identified the duplicated sequences, pax8 -CNS1 and pax2 -CNS1 ( Fig. 1a,b ), which implied the partial conservation of cis -regulatory mechanisms between pax8 and pax2 . This possibility was supported by the recapitulation of pax2 expression by the pax8 enhancers including pax8 -CNS1 ( Fig. 2 ). The pax8 -CNS1 and pax2 -CNS1 were cloned previously from the pufferfish and were shown to have enhancer activity in a transgenic zebrafish assay [23] . As the activity of pax2 -CNS1 has not been examined in tetrapods, it was cloned from X. tropicalis for the present study and used in the transgenic Xenopus assay. The pax2 -CNS1 drove GFP expression from the β -actin basal promoter in all tissues where the pax8 -CNS1 was active ( Fig. 4a , compare with Fig. 2b ), indicating that their pleiotropic enhancer activities are conserved. We note that these expression domains include not only the pax2 -expressing tissues but also the somite and midbrain, which suggests that pax2 also has a silencer(s) somewhere in its regulatory region but the tissue range of this putative pax2 silencer is much more restricted than that for pax8 . 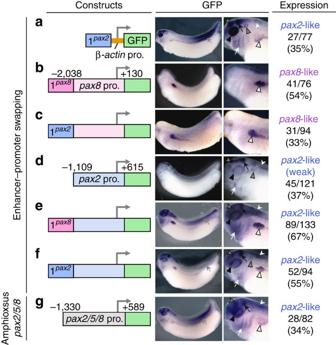Figure 4: Silencer innovation inpax8is crucial for generating divergence in the expression ofpax8andpax2. TransgenicX. laevisembryos were generated with the following GFP constructs. (a) TheX. tropicalis pax2-CNS1 (shown as 1pax2) was linked to the β-actinbasal promoter-GFP cassette. (b,c) TheX. tropicalis pax8proximal promoter (−2038 to +130) was flanked by either theX. tropicalis pax8-CNS1 (b) orpax2-CNS1 (c). (d) The proximal promoter region ofX. tropicalis pax2(−1109 to +615) alone was linked to GFP. (e,f) TheX. tropicalis pax2proximal promoter was flanked by either theX. tropicalis pax8-CNS1 (e) orpax2-CNS1 (f). (g) The amphioxuspax2/5/8promoter (−1330 to +589) was linked to GFP. White, grey and black triangles indicate expression in the pronephros, otic vesicle and eye, respectively. White, grey and black arrows indicate expression in the pharyngeal arches, somites and MHB, respectively. White and grey arrowheads indicate expression in the hindbrain and in an anterior part of the midbrain, respectively. Figure 4: Silencer innovation in pax8 is crucial for generating divergence in the expression of pax8 and pax2 . Transgenic X. laevis embryos were generated with the following GFP constructs. ( a ) The X. tropicalis pax2 -CNS1 (shown as 1 pax2 ) was linked to the β -actin basal promoter-GFP cassette. ( b , c ) The X. tropicalis pax8 proximal promoter (−2038 to +130) was flanked by either the X. tropicalis pax8 -CNS1 ( b ) or pax2 -CNS1 ( c ). ( d ) The proximal promoter region of X. tropicalis pax2 (−1109 to +615) alone was linked to GFP. ( e , f ) The X. tropicalis pax2 proximal promoter was flanked by either the X. tropicalis pax8 -CNS1 ( e ) or pax2 -CNS1 ( f ). ( g ) The amphioxus pax2/5/8 promoter (−1330 to +589) was linked to GFP. White, grey and black triangles indicate expression in the pronephros, otic vesicle and eye, respectively. White, grey and black arrows indicate expression in the pharyngeal arches, somites and MHB, respectively. White and grey arrowheads indicate expression in the hindbrain and in an anterior part of the midbrain, respectively. Full size image Next, we investigated whether the silencer element in the pax8 proximal promoter could limit the enhancer functions of pax8 -CNS1 and pax2 -CNS1 in a similar tissue-specific fashion. To test this possibility, GFP reporter constructs, carrying either pax8 -CNS1 or pax2 -CNS1 with the pax8 proximal promoter (−2038 to +130), were subjected to a transgenic assay. In the resulting embryos, GFP expression from both constructs was restricted to the pronephros, which mostly recapitulated endogenous pax8 expression ( Fig. 4b,c ). We also performed experiments using the pax2 proximal promoter region (−1109 to +615 of X. tropicalis pax2 ) in place of the pax8 proximal promoter. This pax2 promoter in itself drove weak GFP expression in the pax2 -expression domains ( Fig. 4d ). When this pax2 promoter was flanked by the pax8 -CNS1 or pax2 -CNS1, GFP expression mimicked pax2 expression in the pronephros, pharyngeal arches, MHB and hindbrain ( Fig. 4e,f ) in contrast with the experiments using the pax8 promoter. These results indicated that silencer activity uniquely associated with the pax8 proximal promoter is the primary factor generating the divergence of expression between pax8 and pax2 . Finally, we asked whether pax8 acquired the silencer following the WGD event(s), or whether both pax8 and pax2 inherited the element from their common progenitor but only pax2 has lost it. The pleiotropic expression observed for the amphioxus gene, pax2/5/8 , suggests the first scenario [9] . To examine this possibility, a GFP reporter construct carrying the amphioxus pax2/5/8 promoter (−1330 to +589, Supplementary Fig. S5 ) was generated and used in the transgenic assay. This construct drove GFP expression in the eye, pharyngeal arches, MHB, hindbrain and pronephros, and the expression was very similar to that driven by pax8 -CNS1 or pax2 -CNS1 from the pax2 proximal promoter ( Fig. 4g , compare with Fig. 4e,f ). This pleiotropic activity of the pax2/5/8 promoter supports the idea that the silencer is an evolutionary innovation in the pax8 promoter. In this study, we have shown that both pax8 and pax2 retain the ancestral modes of cis -activation involving the duplicated enhancers, and that the innovation of a tissue-specific silencer in pax8 has had a crucial role in generating divergence in the expression of these paralogues. A previous study in teleosts suggested the conservation of the duplicated enhancers between pax8 and pax2 [23] . However, the activities of this and other pax8 enhancers to drive pax2 -like expression and the mechanism for suppressing such pleiotropic activities outside the pax8 -expressing tissues had remained unknown. Sequence analysis identified putative binding motifs of transcriptional repressors, REST (also known as NRSF) [24] , [25] and Nkx [26] , [27] , in the silencer region of X. tropicalis pax8 promoter and its orthologous region of mouse Pax8 , but not in the homologous regions of X. tropicalis pax2 or amphioxus pax2/5/8 ( Supplementary Fig. S6 ). The unique association of these repressor motifs to the pax8 promoter implies their involvement in silencer activity. In our transgenic assay, both the Xenopus and mouse pax8 proximal promoters showed silencer activities but their tissue specificities were slightly different: the Xenopus promoter suppressed expression in the MHB but the mouse promoter did not (compare Figs 3g and 4b ). Given that the Xenopus and mouse pax8 enhancers (CNS1) are both capable of directing expression in the MHB, this difference in the silencer activities might account for the species differences in the MHB expression of Xenopus and mouse pax8 . It has been shown that the thyroid gland expression of pax8 and pax2 also shows species difference: thus, zebrafish expresses both pax8 and pax2 , whereas Xenopus and mouse exclusively express pax2 and pax8 , respectively, in the developing thyroid [12] , [13] , [28] . Although such overlapping or reciprocal expression implies the conservation of thyroid enhancers between pax8 and pax2 and species-specific modification of the silencers, our transgenic experiments did not detect any expression in the thyroid with either pax8 -CNSs or pax2 -CNS1 ( Supplementary Fig. S7 ). Thus, a thyroid enhancer(s) might be present outside these CNSs in the pax8 and pax2 loci, and the involvement of any silencers remains unknown. Given that only one pair of enhancers is conserved between pax8 and pax2 , complementary degeneration likely occurred in some of their duplicated enhancers after the WGD events. The silencer innovation in pax8 promoter occurred either before or after the enhancer degeneration, and these two events have led to the resolution of their duplicated expression in modern vertebrates ( Fig. 5 ). This process may also have involved the innovation of another pax8 enhancer(s) and/or silencer(s), whose presence was suggested by the fosmid reporter assay. Possibly, the duplicated expression of pax8 and pax2 was advantageous for evolution of the kidney and ear but disadvantageous for other tissues. If pax8 and pax2 had inherited monofunctional enhancers rather than pleiotropic ones from their common progenitor, any disadvantages caused by duplication of their expression would have been fully dissolved by degeneration of the enhancers responsible, as predicted by the duplication–degeneration–complementation model. However, because pleiotropic enhancers such as pax8 -CNS1 and pax2 -CNS1 drove both advantageous and disadvantageous expressions, the silencer innovation was necessary to suppress the latter. The redundant regulatory system of pax8 that involves additional enhancers, CNS2–CNS4, with overlapping activities might also have contributed to this silencer innovation by robust protection of the original expression pattern from degenerative mutations. 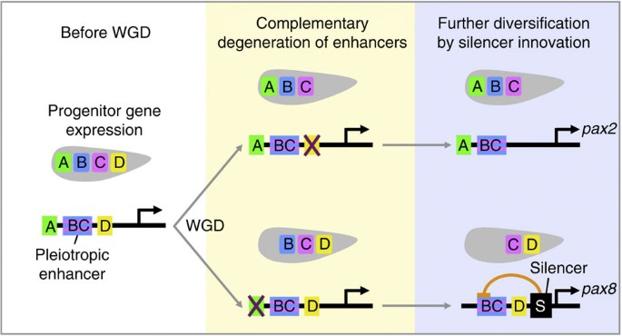Figure 5: A model for the regulatory diversification ofpax2andpax8. To simplify the model,pax5is not depicted. The model is based on a progenitor gene with four expression domains (A, B, C and D) and three enhancers (A, BC and D), where the pleiotropic enhancer, BC, drives expression in both B and C domains (left panel). Following WGD1 and/or WGD2, the complementary loss of enhancers occurs in the duplicated genes: one (pax2) loses the D enhancer and the other (pax8) loses the A enhancer because of degenerative mutations ('×' in the middle panel). Silencer innovation then occurs in the proximal promoter ofpax8(black box 'S'), to allow selective suppression of BC enhancer activity in the B domain (right panel, orange line). Figure 5: A model for the regulatory diversification of pax2 and pax8 . To simplify the model, pax5 is not depicted. The model is based on a progenitor gene with four expression domains (A, B, C and D) and three enhancers (A, BC and D), where the pleiotropic enhancer, BC, drives expression in both B and C domains (left panel). Following WGD1 and/or WGD2, the complementary loss of enhancers occurs in the duplicated genes: one ( pax2 ) loses the D enhancer and the other ( pax8 ) loses the A enhancer because of degenerative mutations ('×' in the middle panel). Silencer innovation then occurs in the proximal promoter of pax8 (black box 'S'), to allow selective suppression of BC enhancer activity in the B domain (right panel, orange line). Full size image The two features present in pax8 enhancers, pleiotropy and redundancy, have been found in the regulation of many developmental genes. For example, Sox10 has three enhancers that drive overlapping expression in four discrete neural tissues [29] , and Sonic hedgehog has two enhancers that drive overlapping expression in the notochord and tegmentum [30] . Recent studies in Drosophila have revealed that such redundant regulation involves 'shadow enhancers', which ensure robust gene expression under adverse environmental or genetic conditions [31] , [32] , [33] . Therefore, the redundant pax8 enhancers might function as shadow enhancers, and silencer innovation could be a common evolutionary escape route for developmental genes that harbour such robust regulatory mechanisms. Genome sequence analysis The 160-kb genomic sequence of the human PAX8 locus (hg18, chr2: 113,675,016–113,835,015) and its orthologous sequences in the mouse (mm9, chr2: 24,262,407–24,415,729), X. tropicalis (xenTro2, scaffold_30: 1,830,001–1,870,000) and Takifugu (fr2, chrUn: 75,566,029–75,596,029) were downloaded from the UCSC Genome Browser [34] . The genomic sequence of the human PAX2 locus (hg18, chr10: 102,287,183–102,677,960) and its orthologous sequences in the mouse (mm9, chr19: 44,638,956–45,020,167), X. tropicalis (xenTro2, scaffold_204: 1,014,773–1,688,046) and Takifugu (fr2, chrUn: 158,920,197–159,034,770) were also downloaded from this genome browser. These sequences were aligned using MultiPipMaker [16] . Sequence alignments of the pax8 -CNS1 and pax2 -CNS1, amphioxus pax2/5/8 promoters, and the pax8 , pax2 and amphioxus pax2/5/8 proximal promoters were generated using ClustalW [35] . Searches for potential transcription factor-binding sites were performed with transcription factor-binding motifs collected from the TRANSFAC and JASPAR databases [36] , [37] . Putative transcription start sites of X. tropicalis pax8 , pax2 , mouse Pax8 and amphioxus pax2/5/8 were predicted with their previously identified complementary DNAs (Genbank accession numbers: NM001079301 , AL969279 , NM011040 and AF053762 , respectively) and an eukaryotic promoter prediction program [38] . Plasmid and fosmid constructs The reporter plasmid, actGFP, carrying a chicken β -actin basal promoter (−55 to +53), was previously described as βGFP [18] . The construct, gloGFP, was generated by replacing the β -actin basal promoter of actGFP with a human β -globin basal promoter (−37 to +12) [20] . Primer sequences used in this study are summarized in Supplementary Table S3 . The CNSs and other promoter regions were cloned from X. tropicalis , mouse or Japanese amphioxus ( Branchiostoma japonicum ) genomic DNA by PCR and verified by sequencing. The sequence of the B. japonicum pax2/5/8 promoter was deposited to GenBank (accession no. JQ902140 ). The reporter constructs carrying the pax2 , pax8 or pax2/5/8 promoters were generated by introducing each fragment into the promoter-less GFP reporter plasmid, pBSSK+EGFP [18] . For generating the pax8 –GFP fosmid construct, a GFP-flpe- kan cassette was introduced in-frame into a X. tropicalis fosmid clone, AOPZ250282 (European Xenopus Resource Centre), using homologous recombination technique [39] . After the recombination, the kan gene used as a selection marker was flipped out from the fosmid by arabinose-induced Flpe recombinase [40] . Transgenic reporter assay Transgenic Xenopus embryos were generated by a sperm nuclear transplantation method with oocyte extracts [17] , [41] . The manipulated embryos were cultured until the tailbud stages, and all normally developed embryos were subjected to in situ hybridization to examine their GFP expression with maximum sensitivity [18] . The frequency of GFP expression varied depending on constructs, egg quality and preparation of the oocyte extracts. However, within any GFP-positive group, more than 80% showed an expression pattern consistent with the representative examples, and the remainder showed non-reproducible ectopic expression ( Supplementary Fig. S2 and Supplementary Table S1 ). How to cite this article: Ochi, H. et al . Evolution of a tissue-specific silencer underlies divergence in the expression of pax2 and pax8 paralogues. Nat. Commun. 3:848 doi: 10.1038/ncomms1851 (2012).